Interfacial control of oxygen vacancy doping and electrical conduction in thin film oxide heterostructures Oxygen vacancies in proximity to surfaces and heterointerfaces in oxide thin film heterostructures have major effects on properties, resulting, for example, in emergent conduction behaviour, large changes in metal-insulator transition temperatures or enhanced catalytic activity. Here we report the discovery of a means of reversibly controlling the oxygen vacancy concentration and distribution in oxide heterostructures consisting of electronically conducting In 2 O 3 films grown on ionically conducting Y 2 O 3 -stabilized ZrO 2 substrates. Oxygen ion redistribution across the heterointerface is induced using an applied electric field oriented in the plane of the interface, resulting in controlled oxygen vacancy (and hence electron) doping of the film and possible orders-of-magnitude enhancement of the film's electrical conduction. The reversible modified behaviour is dependent on interface properties and is attained without cation doping or changes in the gas environment. The discoveries of a wide range of remarkable behaviours in thin film oxide heterostructures have led to intense interest in their synthesis and characterization. Oxygen vacancy concentrations exceeding bulk levels near surfaces and interfaces have recently been cited as instrumental in controlling these behaviours. For example, large changes in electrical resistance associated with metal-insulator transitions [1] , [2] or resistive switching behaviour [3] , [4] have been linked to increased oxygen vacancy concentrations in thin film heterostructures. Magnetism in thin film heterostructures of bulk non-magnetic materials [5] , [6] has been attributed to the presence of oxygen vacancies near interfaces [7] , [8] , [9] , [10] , and catalytic activity of oxide heterostructures has been explained by enhanced interfacial oxygen vacancy concentrations [11] , [12] , [13] , [14] , [15] , [16] . Also, localized metallic conduction has been reported near heterointerfaces between bulk oxide insulators (e.g., LaAlO 3 /SrTiO 3 ) [17] . While the origin of this remarkable conduction behaviour is the subject of continuing debate, several authors have concluded that it is caused by oxygen vacancy doping of SrTiO 3 substrates during thin film deposition [18] , [19] , [20] , [21] , [22] . These examples demonstrate the importance of being able to manipulate oxygen vacancies to achieve emergent behaviour, motivating the exploration of new ways to control vacancy concentrations and distributions in oxide thin film heterostructures. In this study, we investigated the possibility of using electric fields to control oxygen vacancies in model thin film heterostructures, primarily epitaxial thin films of In 2 O 3 grown on (001) and (111) surfaces of Y 2 O 3 -stabilized ZrO 2 (YSZ). In the following, we show that, when a small in-plane electric field is applied to In 2 O 3 -on-YSZ heterostructures, the measured electrical conductance rises dramatically, in some cases by more than two orders-of-magnitude. The question thus arises: How do electrons and ions in these heterostructures interact to produce this remarkable phenomenon? We show that the effect arises from the response to resistances that develop at the electrodes following application of the in-plane field. Field-induced conductance increase Epitaxial In 2 O 3 films were deposited on single crystal (001) YSZ, (111) YSZ or (001) MgAl 2 O 4 substrates. The <2% misfit strain between bixbyite-structured In 2 O 3 and fluorite-structured YSZ enables the growth of epitaxial single crystal films with a cube-on-cube orientation relationship between the film and substrate [23] , [24] , [25] . In 2 O 3 is an oxide semiconductor, exhibiting n-type conductivity [26] , [27] (see Supplementary Fig. 1 and Supplementary Note 1 ). In contrast, YSZ is a fast oxygen ion conductor with negligible electronic conductivity [28] . Oxygen ions in the ionically conducting YSZ substrate will migrate in an electric field, with oxygen vacancies moving towards the negative electrode. Oxygen ions enter YSZ at triple phase boundaries at the negative electrode according to , which is written using Kröger-Vink notation [29] , where indicates an oxygen vacancy with a +2 charge, e′ is an electron and is an oxygen ion with a formal −2 valence sitting in an oxygen lattice site. Oxygen exits the sample at the positive electrode by the reverse reaction. Electrical characterization was performed on samples with the electrode geometry shown in Fig. 1 . We monitored the conductance response when small DC fields were applied in the plane of the film by flowing current between electrodes 1 and 7 while monitoring the voltage using a pair of electrodes on the surface of the film (shown as 5 and 6 in Fig. 1 ). Surprisingly, all samples grown on YSZ that were exposed to small DC fields showed a monotonic rise in conductance with time, such as is shown in Fig. 2 . In this particular case, with a field of ∼ 4 V cm −1 applied, the conductance increased by a factor of nearly 200 relative to the starting (zero field) value. 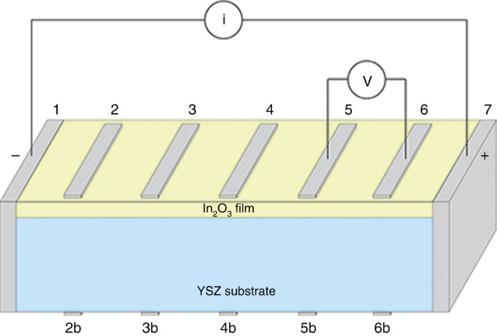Figure 1: Sample schematic. Equally spaced Pt parallel line electrodes (voltage pick-offs) were sputter-deposited through a shadow mask on the films (numbered 2–6) and, for some samples, on the other surface of the YSZ substrate (2b-6b). The current electrodes (numbered 1 and 7) were Ag or Pt paint. Figure 1: Sample schematic. Equally spaced Pt parallel line electrodes (voltage pick-offs) were sputter-deposited through a shadow mask on the films (numbered 2–6) and, for some samples, on the other surface of the YSZ substrate (2b-6b). The current electrodes (numbered 1 and 7) were Ag or Pt paint. 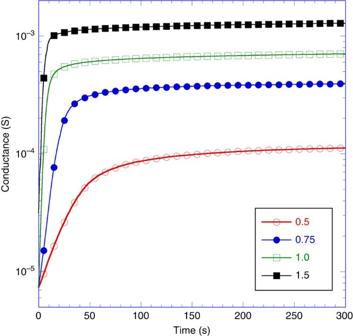Figure 2: Field-induced electrical conductance increase. Time-dependent increases in conductance were observed at different measurement voltages. VoltageV23was held constant at the values indicated in the legend (in Volts), while flowing current between electrodes 1 and 7. The electrode configuration is shown inFig. 1. The conductance is enhanced by a factor of 190 at the highest voltage (field) shown. The measurements were taken at 370 °C, with the sample equilibrated atpO2=150 torr. Full size image Figure 2: Field-induced electrical conductance increase. Time-dependent increases in conductance were observed at different measurement voltages. Voltage V 23 was held constant at the values indicated in the legend (in Volts), while flowing current between electrodes 1 and 7. The electrode configuration is shown in Fig. 1 . The conductance is enhanced by a factor of 190 at the highest voltage (field) shown. The measurements were taken at 370 °C, with the sample equilibrated at p O 2 =150 torr. Full size image The conductance enhancement was found to be reversible, with the conductance returning to approximately the original value after removal of the field. The relative change in conductance was observed to increase with decreasing film thickness (see Supplementary Table 1 ). This indicates that the field-induced conduction enhancement is localized to a region in the films near the film/substrate heterointerface. Responses of interfaces to applied fields Further experiments were carried out to determine the mechanism responsible for the observed field-induced conductance increases. These measurements clearly demonstrate that the dramatic enhancement of the sample conductance is determined by the response of multiple interfaces in the heterostructure to the application of small electric fields. There are five relevant interfaces in the heterostructure. In addition to the planar YSZ/In 2 O 3 interface, Ag/YSZ and Ag/In 2 O 3 interfaces (or Pt/YSZ and Pt/In 2 O 3 interfaces), at both positive and negative electrodes, must be considered. Pt/In 2 O 3 interfaces at the voltage pickoffs do not contribute to the observed behaviour, since a four-electrode configuration is used and pick-off voltages are measured with a high input impedance voltmeter. When a DC field is applied between the end electrodes (electrodes 1 and 7 in Fig. 1 ), a voltage profile is established laterally across the sample. If there are no contact resistances, and samples are homogeneous, the profiles across the In 2 O 3 and YSZ are identical. However, if contact resistances at the electrode/film and electrode/substrate interfaces differ, the lateral voltage profile across the In 2 O 3 film can be different from that across the YSZ substrate. This can happen because YSZ is an ionic conductor and In 2 O 3 is an electronic conductor. 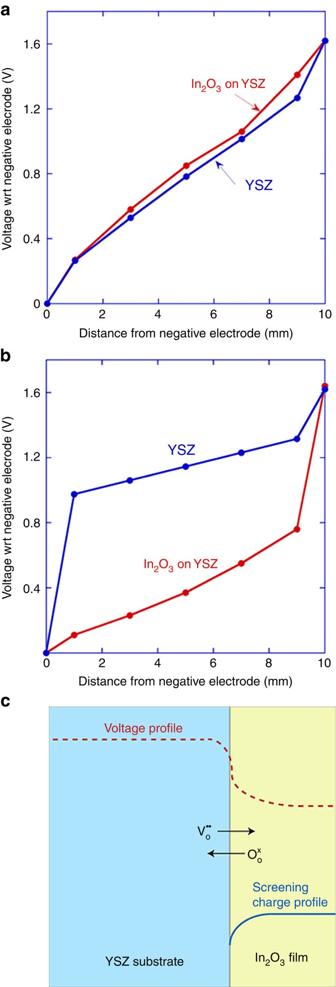Figure 3: Voltage profiles. (a) Initial voltage profile across a bare YSZ substrate compared with the profile across a 51 nm thick In2O3-on-YSZ sample when a 1.6 volt battery is connected to electrodes 1 and 7 at 330 °C (electrode configuration shown inFig. 1). Minimal contact resistances are present initially. (b) The voltage profiles after 5 min (at steady state) for the same two samples. For the bare YSZ substrate, a large contact resistance has developed at the negative electrode (where oxygen entry occurs). A smaller contact resistance appears at the positive electrode (oxygen exit). A Schottky-type resistance appears at the positive electrode of the In2O3-on-YSZ sample. As a result of these resistances, a voltage drop develops between YSZ and the In2O3film, with the substrate at a higher potential than the film. (c) The voltage profile that develops across the In2O3/YSZ interface causes oxygen ions to move across the interface from In2O3to YSZ. A screening charge appears in the In2O3film near the interface. This interfacial electron doping increases the conductivity of the In2O3. In the YSZ, charge neutrality is maintained by mobile excess oxygen ions moving away from the interface. Figure 3a shows measured voltage profiles across a bare substrate and a thin film heterostructure, with Pt end electrodes, at time t =0, when the DC field is first applied. Figure 3b shows the profiles across the same two samples after relaxation to steady state has occurred. The initial profiles in Fig. 3a are nearly identical, indicating that all contact resistances are similar and small at time zero, when the voltage is first applied. However, at steady state, the profiles shown in Fig. 3b have dramatically diverged. A large resistance has developed at the negative Pt electrode/YSZ interface, where oxygen entry occurs. The resistance at the positive Pt electrode/YSZ interface, where oxygen exit occurs, shows very little change with time. At the same time, a large resistance develops at the positive Pt electrode/In 2 O 3 interface. No significant resistance develops at the negative Pt electrode/In 2 O 3 interface. Supplementary Figs 2 and 3 show the time development of similar contact resistances when the end electrodes are Ag rather than Pt. Figure 3: Voltage profiles. ( a ) Initial voltage profile across a bare YSZ substrate compared with the profile across a 51 nm thick In 2 O 3 -on-YSZ sample when a 1.6 volt battery is connected to electrodes 1 and 7 at 330 °C (electrode configuration shown in Fig. 1 ). Minimal contact resistances are present initially. ( b ) The voltage profiles after 5 min (at steady state) for the same two samples. For the bare YSZ substrate, a large contact resistance has developed at the negative electrode (where oxygen entry occurs). A smaller contact resistance appears at the positive electrode (oxygen exit). A Schottky-type resistance appears at the positive electrode of the In 2 O 3 -on-YSZ sample. As a result of these resistances, a voltage drop develops between YSZ and the In 2 O 3 film, with the substrate at a higher potential than the film. ( c ) The voltage profile that develops across the In 2 O 3 /YSZ interface causes oxygen ions to move across the interface from In 2 O 3 to YSZ. A screening charge appears in the In 2 O 3 film near the interface. This interfacial electron doping increases the conductivity of the In 2 O 3 . In the YSZ, charge neutrality is maintained by mobile excess oxygen ions moving away from the interface. Full size image Electrochemical reactions associated with oxygen entry and exit are likely to be responsible for the time-dependent increases in resistance at the YSZ/metal electrode/environment triple junctions when a DC potential is applied. For example, time-dependent changes in the polarization resistance at Pt electrode/YSZ electrolyte/environment triple junctions have been reported in numerous studies and have often been linked with formation of nonstoichiometric PtO x at the interface when a potential is applied [30] , [31] , [32] , [33] . This field-driven PtO x formation may impede the oxygen exchange reactions that occur at the triple junctions [34] , altering the contact resistances. While the electrochemistry of Ag/YSZ junctions in oxidizing environments has not been as extensively studied as Pt/YSZ, a similar impediment to oxygen exchange would be expected to occur if Ag electrodes in contact with the YSZ are oxidized at the triple junctions when a field is applied. The observed rectifying behaviour of the positive and negative electrode junctions with the film ( Supplementary Fig. 3 ) may be associated with the formation of a Schottky barrier at the positive electrode/In 2 O 3 interface, which has been reported to develop between In 2 O 3 films and Pt electrodes when oxygen vacancies are eliminated from the region of the heterointerface [35] . In the current experiment, oxygen ions migrate towards the positive current electrode under the influence of the applied field, eliminating oxygen vacancies from the In 2 O 3 film near the interface with the positive current electrode. Voltage across the film/substrate interface As a result of the changes in the interfacial resistances (primarily at the negative electrode/YSZ interface and at the positive electrode/In 2 O 3 interface), which develop with field exposure, a substantial voltage drop appears between the YSZ substrate and the In 2 O 3 film. The voltage drop is concentrated at the In 2 O 3 /YSZ interface, where ionic and electronic conductors meet, as illustrated in Fig. 3c . This component of the field, oriented normal to the interface, moves electrons in In 2 O 3 and oxygen vacancies in YSZ towards the interface and provides a driving force to move oxygen ions from the film to the substrate. Enhanced electron doping of the In 2 O 3 occurs within a relatively short distance, that is, a screening length of ∼ 10 nm from the interface, as discussed in Supplementary Note 2 . While the detailed physical processes controlling the electrochemistry at the contacts remain under active investigation, for our purposes it is sufficient to monitor the development of the contact resistances following application of a DC voltage. Consideration of the time-dependent behaviour appears in Supplementary Figs 4 and 5 and Supplementary Note 1 . As seen in Fig. 4 , the development of the potential across the In 2 O 3 /YSZ interface was confirmed by directly measuring the voltage between pairs of electrodes on the top and bottom surfaces of a sample as a function of time while again flowing current between electrodes 1 and 7. The voltage across the In 2 O 3 /YSZ interface was observed to increase from zero with time of field application, with YSZ at a higher potential than In 2 O 3 , consistent with the measurements shown in Fig. 3b . 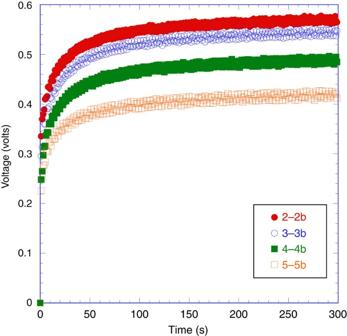Figure 4: Development of voltage across the film/substrate interface. The voltage drop measured between the film surface and the back surface of the substrate at four positions on a sample when an in-plane current of 5 × 10−5Amps is imposed between electrodes 1 and 7 (seeFig. 1for electrode configuration). The legend denotes the pairs of top/bottom electrodes used for each measurement. Measurements were taken at 370 °C, with the sample equilibrated atpO2=1.5 torr. Figure 4: Development of voltage across the film/substrate interface. The voltage drop measured between the film surface and the back surface of the substrate at four positions on a sample when an in-plane current of 5 × 10 −5 Amps is imposed between electrodes 1 and 7 (see Fig. 1 for electrode configuration). The legend denotes the pairs of top/bottom electrodes used for each measurement. Measurements were taken at 370 °C, with the sample equilibrated at p O 2 =1.5 torr. Full size image Since a DC in-plane electric field imposes a voltage in a direction normal to the film/substrate interface, which drives oxygen ions from the In 2 O 3 film into the YSZ substrate, we investigated whether a similar doping effect might be achieved by directly applying a voltage across the YSZ/In 2 O 3 heterointerface. 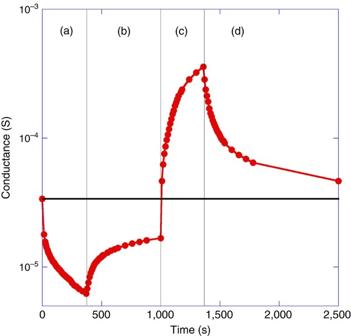Figure 5: Applying a voltage across the film/substrate interface. Measurements of the average conductance between electrodes 1 and 7, plotted versus time when a voltage is applied between electrodes 4 and 4b using a battery (seeFig. 1for the electrode configuration). Region (a): Applying 1.6 V, with the film at a higher potential than the substrate, moves oxygen ions from YSZ into the In2O3. This reduces the oxygen vacancy doping of the film, thus reducing the measured conductance. Region (b): When the battery is open-circuited, the conductance relaxes towards the initial value as the film’s oxygen vacancy concentration returns to the equilibrium value determined by the temperature andpO2. Region (c): Applying 1.6 V, with the substrate at a higher potential than the film, moves oxygen ions from In2O3into the YSZ. This oxygen vacancy dopes the film, thus increasing the measured conductance. Region (d): Removing the battery again results in the measured conduction relaxing towards the starting value as the film oxygen vacancy concentration returns to that set by the temperature andpO2. The measurements were taken at 330 °C withpO2=1.5 torr. Figure 5 shows measurements when a voltage is applied between electrodes on the top and bottom surfaces of the sample using a battery, while the average conductance in the in-plane direction is measured between the end electrodes. We see that, consistent with our other observations, the average conductance increases when the substrate is at a higher potential than the substrate, while the conductance decreases when the voltage direction is reversed to place the substrate at a lower potential than the film. Figure 5: Applying a voltage across the film/substrate interface. Measurements of the average conductance between electrodes 1 and 7, plotted versus time when a voltage is applied between electrodes 4 and 4b using a battery (see Fig. 1 for the electrode configuration). Region (a): Applying 1.6 V, with the film at a higher potential than the substrate, moves oxygen ions from YSZ into the In 2 O 3 . This reduces the oxygen vacancy doping of the film, thus reducing the measured conductance. Region (b): When the battery is open-circuited, the conductance relaxes towards the initial value as the film’s oxygen vacancy concentration returns to the equilibrium value determined by the temperature and p O 2 . Region (c): Applying 1.6 V, with the substrate at a higher potential than the film, moves oxygen ions from In 2 O 3 into the YSZ. This oxygen vacancy dopes the film, thus increasing the measured conductance. Region (d): Removing the battery again results in the measured conduction relaxing towards the starting value as the film oxygen vacancy concentration returns to that set by the temperature and p O 2 . The measurements were taken at 330 °C with p O 2 =1.5 torr. Full size image Development of a conductance gradient Figures 3b and 4 also show that the voltage drop between YSZ and the In 2 O 3 film is larger near the negative current electrode than it is near the positive current electrode, suggesting that a conductance gradient will appear in the film. 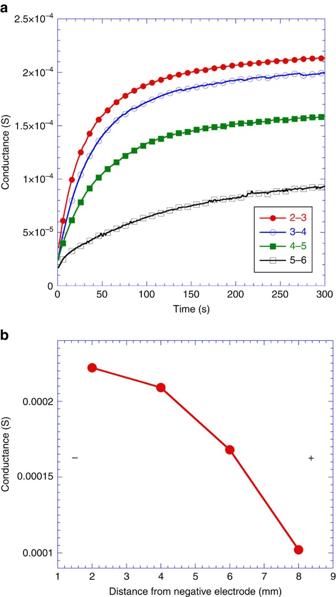Figure 6: Evidence of a conduction gradient. (a) Time dependence of conductance measured between adjacent pairs of voltage pick-off electrodes (denoted in the legend), with a constant current of 5E-5 amps flowing between electrodes 1 and 7 (seeFig. 1for electrode configuration). Measurements were taken at 370 °C, with the sample equilibrated atpO2=1.5 torr. (b) Conductance as a function of position on the sample, at steady state. The conductance is largest near the negative current electrode and shows a gradient across the sample. Figure 6a confirms this, showing the time dependence of the average conductance between adjacent electrodes under constant current conditions. The largest conduction enhancement at steady state is observed when the voltage pick-off electrodes used are closest to the negative current electrode. Figure 6b shows the corresponding field-enhanced conductance values at steady state, as a function of position on the sample. As expected, the conductance is largest near the negative electrode and shows a gradient across the sample. Figure 6: Evidence of a conduction gradient. ( a ) Time dependence of conductance measured between adjacent pairs of voltage pick-off electrodes (denoted in the legend), with a constant current of 5E-5 amps flowing between electrodes 1 and 7 (see Fig. 1 for electrode configuration). Measurements were taken at 370 °C, with the sample equilibrated at p O 2 =1.5 torr. ( b ) Conductance as a function of position on the sample, at steady state. The conductance is largest near the negative current electrode and shows a gradient across the sample. Full size image We note that electric field-induced polarization has been observed to occur in many different mixed oxide conductors (that is, oxides that exhibit both ionic and electronic conduction), a manifestation of the well-known Hebb-Wagner polarization mechanism [36] , [37] . Hebb-Wagner polarization occurs in mixed electron/ion conductors exposed to a DC field when ionic conduction is blocked by a current electrode. Resultant polarization of the mobile ions may in turn locally alter the electronic conductivity, producing an electronic conductivity gradient. Hebb-Wagner polarization is not observed in In 2 O 3 or YSZ because these oxides are not mixed conductors. While, similar to Hebb-Wagner behaviour, we observe in-plane polarization (development of a conductivity gradient) when applying an in-plane DC field, the polarization mechanism observed here results from the development of different electric field profiles in the substrate and film, which is not a characteristic of the Hebb-Wagner mechanism. The electrical behaviour of the heterostructure, at steady state, is approximately represented by the equivalent circuit shown in Supplementary Fig. 6 and discussed in Supplementary Note 3 . Since the measured field-induced conductance enhancement depends on the distance of the voltage pick-off electrodes from the negative current electrode, it is expected that reversing the current direction, which changes that spacing and also reverses the conduction gradient, will result in a different steady state conductance being attained (unless the pick-off electrodes are symmetrically located with respect to the current electrodes, in which case the distance of the pick-off electrodes from the negative current electrode is not changed by reversing the current direction). 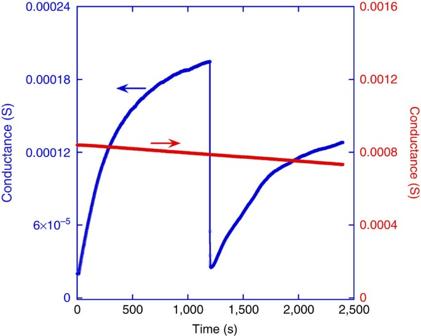Figure 7: Comparison of the behaviour of different substrates. Conductance versus time for In2O3/YSZ (blue,) and In2O3/MgAl2O4(red) samples, under constant current conditions. The field was applied att=0, and the field direction was reversed for both samples att=1,200 s. Transient behaviour was observed for the In2O3/YSZ sample, with the conductance evolving towards a different steady-state conductance for the two current directions. This behaviour occurs because the voltage pick-off electrodes are asymmetrically located with respect to the current electrodes. Since MgAl2O4is not a fast oxygen ion conductor, the field application and reversal had no effects on the measured conductance of the In2O3/MgAl2O4sample. Both samples were measured at 330 °C withpO2=1.5 torr. Figure 7 shows measurements that confirm this behaviour. The current-reversal observations shown in Fig. 7 also rule out sample resistive heating as a cause of the field-induced enhanced conductance. Resistive heating would be independent of current direction, always acting to increase the conductance, and would not produce a gradient. Figure 7: Comparison of the behaviour of different substrates. Conductance versus time for In 2 O 3 /YSZ (blue,) and In 2 O 3 /MgAl 2 O 4 (red) samples, under constant current conditions. The field was applied at t =0, and the field direction was reversed for both samples at t =1,200 s. Transient behaviour was observed for the In 2 O 3 /YSZ sample, with the conductance evolving towards a different steady-state conductance for the two current directions. This behaviour occurs because the voltage pick-off electrodes are asymmetrically located with respect to the current electrodes. Since MgAl 2 O 4 is not a fast oxygen ion conductor, the field application and reversal had no effects on the measured conductance of the In 2 O 3 /MgAl 2 O 4 sample. Both samples were measured at 330 °C with p O 2 =1.5 torr. Full size image Importance of the substrate and the film/substrate interface Constant current measurements of conductance, with reversal of current direction, are also shown in Fig. 7 for an In 2 O 3 -on-MgAl 2 O 4 sample. While the conductance of the In 2 O 3 film grown on a MgAl 2 O 4 substrate was observed to drift slightly with time due to slow equilibration of the sample under the temperature and oxygen partial pressure conditions used, no change in conductance was observed in response to application of a DC field, nor was a change in conductance observed when the field direction was reversed. These observations demonstrate that the substrate has a profound effect in determining whether field-induced changes in conduction occur, both in establishing the voltage component normal to the heterointerface that provides the driving force for ion motion, and in serving as a source/sink of mobile oxygen vacancies/ions. We hypothesize that In 2 O 3 /MgAl 2 O 4 heterostructures do not show field-induced conduction enhancement because the substrate in this case is not a fast oxygen ionic conductor with a large oxygen vacancy concentration. Since oxygen transport across the In 2 O 3 /YSZ interface is essential to the mechanism described here, we investigated the detailed structure and thermodynamics of the interface using first-principles calculations. In particular, we determined relative oxygen vacancy formation energies near the interface to evaluate the feasibility of the migration of oxygen vacancies into the In 2 O 3 film from the YSZ substrate. We considered the (001) In 2 O 3 /YSZ and In 2 O 3 /ZrO 2 interfaces with atomic stacking normal to the interface that alternates between cation and oxygen planes, with a shared oxygen plane at the interface. Models were considered with different oxygen occupation of the interface plane, from O-deficient to O-rich (see Methods and Supplementary Figs 7 and 8 ). As seen in Fig. 8a , over a wide range of chemical potentials and corresponding T and p O 2 conditions, the formation energy of oxygen-deficient (001) In 2 O 3 /ZrO 2 interfaces is predicted to be lower than the formation energies of vacancies in either bulk material (6.06 eV for ZrO 2 and 4.05 eV for In 2 O 3 ). The vacancy formation energy is possibly reduced at the interface compared with bulk because of the different oxygen stoichiometry and Madelung field on either side of the interface. Bulk ZrO 2 has 16 O ions per plane and bulk In 2 O 3 has 12 O ions per plane in the supercell, while our calculations indicate that the favourable interface oxygen occupation is close to the bulk In 2 O 3 value. This is consistent with the fact that In serves as a dopant in ZrO 2 compensated by oxygen vacancies. 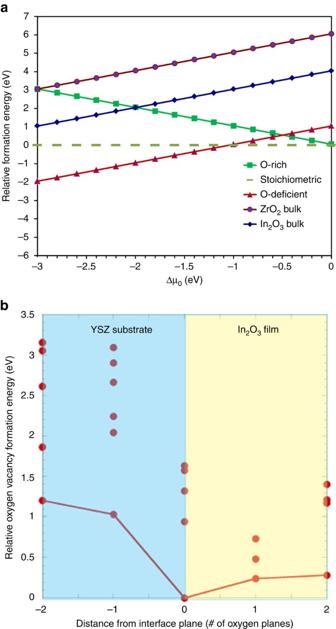Figure 8: Oxygen vacancy formation energies. (a) Relative formation energy per oxygen vacancy for several interface configurations and bulk vacancies in ZrO2and In2O3as a function of oxygen chemical potential relative to molecular oxygen. The zero energy reference is the corresponding stoichiometric structure. (b) On the basis of first-principles calculations, the formation energy associated with adding an oxygen vacancy to a YSZ-In2O3supercell is predicted to be significantly lower for sites in the interface plane or adjacent to the interface in the In2O3film than for sites in the YSZ substrate. Energies for multiple possible sites for an oxygen vacancy within each plane are shown. Points connected with a line correspond to the lowest energy positions of the vacancy in each plane. The formation energy values are relative to the energy of the lowest energy site in the heterostructure. Figure 8: Oxygen vacancy formation energies. ( a ) Relative formation energy per oxygen vacancy for several interface configurations and bulk vacancies in ZrO 2 and In 2 O 3 as a function of oxygen chemical potential relative to molecular oxygen. The zero energy reference is the corresponding stoichiometric structure. ( b ) On the basis of first-principles calculations, the formation energy associated with adding an oxygen vacancy to a YSZ-In 2 O 3 supercell is predicted to be significantly lower for sites in the interface plane or adjacent to the interface in the In 2 O 3 film than for sites in the YSZ substrate. Energies for multiple possible sites for an oxygen vacancy within each plane are shown. Points connected with a line correspond to the lowest energy positions of the vacancy in each plane. The formation energy values are relative to the energy of the lowest energy site in the heterostructure. Full size image We also compared formation energies of an extra oxygen vacancy in different locations of the interface region of a (001) In 2 O 3 /YSZ heterostructure (see Methods and Supplementary Fig. 8 ) to provide insight into the feasibility of an electric field causing oxygen vacancies to migrate from YSZ to the In 2 O 3 side of the interface region. As seen in Fig. 8b , it is energetically favourable for oxygen vacancies in their lowest energy configurations to move from an oxygen plane in YSZ near the interface to the interface plane or an adjacent oxygen plane in the In 2 O 3 film. This will increase the vacancy concentration in In 2 O 3 , consistent with the experimentally observed doping effect. The predicted localization of vacancies to the In 2 O 3 /YSZ interface region is also consistent with the experimentally observed film thickness-dependent behaviour discussed above. The controllable dynamic doping achieved with application of a small lateral (or vertical) electric field demonstrated in this study should be possible in a wide variety of heterostructures. For example, we have also observed similar DC field-induced electrical conduction enhancement in a heterostructure consisting of an epitaxial WO 3 film grown on (001) YSZ ( Supplementary Fig. 9 ). If the heterostructure consists of a film that can be electronically doped by a mobile ion in the substrate, controllable field-driven conductivity should generally be possible. Controllable dynamic doping of the carriers in the electronic conductor can be achieved reversibly, without cation doping or changing the gas environment in contact with the sample, by simply passing a current through the sample parallel to the heterointerface if the field profile in the ionically conducting substrate differs from the profile in the electronically conducting film. This requires that electrode contact resistances in film and substrate are dissimilar, a condition commonly satisfied. While we have focused in this study on using oxygen vacancy doping to control electrical conduction behaviour in a model thin film heterostructure, we expect that similar heterostructures can be designed and synthesized to control other types of behaviours via oxygen stoichiometry control using small electric fields. The approach of using in-plane electric fields to vary oxygen stoichiometry in heterostructures, which consist of a fast oxygen ion conductor with an electronically conducting functional oxide in a thin film, thus provides a new and unexplored opportunity to tune properties and achieve emergent behaviour. Experimental procedures Epitaxial In 2 O 3 films with thicknesses ranging from 4 to 75 nm were deposited by RF sputtering on single crystal (001) or (111) YSZ substrates and on (001) MgAl 2 O 4 substrates with dimensions 1 × 1 cm 2 × 1 mm thickness. The substrate temperature was typically 800 °C, and typical growth rates were approximately 10 nm per hour. Sample thickness was characterized using x-ray reflectivity. X-ray diffraction indicated that the films had the expected cube-on-cube orientation relationship (see Supplementary Fig. 10 and Supplementary Note 4 ). An epitaxial 20 nm thickness WO 3 film was deposited on (001) YSZ, also by RF sputter deposition. Samples had parallel line Pt electrodes sputter-deposited through a shadow mask onto the film surfaces and, in some cases, on the back surface of the substrate, as shown in Fig. 1 . End electrodes were applied using Ag or Pt paint. Most measurements were taken using samples with Ag-painted end electrodes, since bonding of the paint to the sample was generally more reliable (less flaking and measurements were less noisy). Electrical measurements were taken using an environmental probe station, at controlled T and p O 2 . Mass flow controllers were used to mix Ar and O 2 gases to achieve the desired p O 2 , at a total chamber pressure of 150 torr. The measurements were taken at p O 2 =1.5 torr, unless otherwise indicated, at temperatures between 300 and 400 °C. DC fields were applied through Pt-coated probe tips in contact with the sample electrodes, using a Keithley Model 2400 source metre. Conduction measurements were typically taken in four-point geometry, with driving current between the end electrodes and conductance measured between a pair of voltage pick-off electrodes on the film surface, under either fixed voltage or fixed current conditions. Contact resistances were measured using a three-electrode geometry with end electrodes 1 and 7 serving as the current source/sink electrodes, with voltage pickoffs at electrodes 1 and 2, or 6 and 7 ( Fig. 1 ). Resistances between electrodes 1 and 2 or between 6 and 7 (10% of total sample resistance) were included in the 3-electrode measurements. Measurements of the voltage across the In 2 O 3 /YSZ heterointerface were taken by establishing a fixed current between the end electrodes ( Fig. 1 ), while monitoring the voltage between one electrode on the film surface and another electrode, directly beneath, on the backside of the substrate. Computational studies Computational studies used density functional theory within the generalized gradient approximation as implemented in VASP [38] , [39] , with Perdew-Wang exchange-correlation functionals [40] and Projected Augmented Wave potentials [41] . Periodic supercell configurations were analysed, with two interfaces per supercell. Each interface has a shared plane of oxygen ions. As seen in Supplementary Fig. 7 , two configurations were considered: (1) a flat In 2 O 3 cation plane adjacent to the interface, with In ions occupying two sites (8b and 24d), and (2) a buckled In 2 O 3 cation plane adjacent to the interface, with In atoms only occupying 24d sites. In 2 O 3 -ZrO 2 supercells contained three layers of ZrO 2 and five layers of In 2 O 3 (with eight cations in each layer). Structural minimization was performed allowing all the atoms and the supercell in the (001) direction to relax, while keeping the other two dimensions fixed at the bulk value. In 2 O 3 -YSZ supercells comprised five layers of YSZ and five layers of In 2 O 3 . Each YSZ cation layer contained six Zr ions and two Y ions, corresponding to a YSZ stoichiometry equivalent to 6ZrO 2 –Y 2 O 3 . Y ions were distributed in the cell following the approach of a previous computational study [42] . Data availability The data that support the findings of this study are available from the corresponding author upon request. How to cite this article: Veal, B. W. et al . Interfacial control of oxygen vacancy doping and electrical conduction in thin film oxide heterostructures. Nat. Commun. 7:11892 doi: 10.1038/ncomms11892 (2016).